Engineering hybrid nanotube wires for high-power biofuel cells Poor electron transfer and slow mass transport of substrates are significant rate-limiting steps in electrochemical systems. It is especially true in biological media, in which the concentrations and diffusion coefficients of substrates are low, hindering the development of power systems for miniaturized biomedical devices. In this study, we show that the newly engineered porous microwires comprised of assembled and oriented carbon nanotubes (CNTs) overcome the limitations of small dimensions and large specific surface area. Their improved performances are shown by comparing the electroreduction of oxygen to water in saline buffer on carbon and CNT fibres. Under air, and after several hours of operation, we show that CNT microwires exhibit more than tenfold higher performances than conventional carbon fibres. Consequently, under physiological conditions, the maximum power density of a miniature membraneless glucose/oxygen CNT biofuel cell exceeds by far the power density obtained for the current state of art carbon fibre biofuel cells. Increasing low current densities and enhancing mass transport are key challenges in engineering bioelectrochemical materials for sensors and miniature biofuel cells (BFCs), especially in physiological solutions in which concentrations (<0.5 mM) and diffusion coefficients of substrates are very low (<5×10 −5 cm −2 s −1 ). Electrode material and design are critical in addressing such challenges. Different forms of carbon are widely used as electrode base materials because of their chemical stability and good electrical conductivity. It is even more promising when carbon nanotubes (CNTs) are used. CNT electrodes have a particularly high specific surface area enhancing current densities [1] , [2] , [3] , [4] , [5] , [6] , [7] , [8] , [9] . However, the coating of macroelectrodes with CNTs does not allow for faster mass transport. Transport limitations are, however, reduced in microelectrodes with diameters smaller than the diffusion length of their reactants [10] . Radial diffusion allows for faster mass transport compared with semi-infinite planar electrodes. The engineering of new porous and hybrid microwires would be the ideal combination for achieving large surface area and fast mass transport. Electroreduction of oxygen to water is chosen as a key test to validate this concept. This reaction is of great importance as it usually determines the operating voltage and thereby the efficiency of various devices such as air electrodes and BFCs [11] . Platinum has been the reference catalyst for oxygen reduction for more than a century. Nevertheless, it has some drawbacks (large overpotential, deactivation), and new types of electrodes are currently being explored [12] , [13] . Modified carbon fibre (CF) electrodes with bioelectrocatalysts have been shown to operate at overpotentials well below that of platinum [14] . However, they have only a small specific surface and their operational half-lives are only of a few weeks. It is shown here that the engineering of new porous and hybrid microfibres made of oriented and biofunctionalized CNTs allows for particularly high current densities and small overpotential. They are optimized for oxygen reduction and BFC applications, with glucose oxidase (GOx) as the anodic bioelectrocatalyst and bilirubin oxidase (BOD) as the cathodic one ( Fig. 1a ). BFCs are of interest because these could power, in the near future, sensor transmitters that could broadcast, for example, the local glucose concentration, relevant to diabetes management [15] . Nanotube-based glucose/oxygen BFC using GOx and BOD with low-power density have been reported earlier [16] , [17] , [18] , [19] , [20] , [21] , [22] CNT-based electrodes are usually made from dispersions in organic solvent that are drop casted onto electrode surfaces. The power density generated by such devices can range from 1 to 53.9 μW cm −2 for the most efficient devices [17] , [23] . Recently, high-power membrane BFCs haves also been reported to generate 1.45 mW cm −2 at 0.3 V [24] . The elaboration of high-power membraneless BFC is a critical feature for future applications, as membraneless devices can be miniaturized. However, the engineering of membraneless BFCs is challenging because it requires the electrodes to be structured to ensure that the mass transport of reactants and products is not impeded and that all enzymes are electronically and efficiently connected to electrodes. 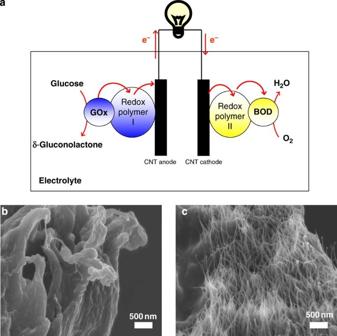Figure 1: Schematic of the biofuel cell and scanning electron micrographs of CNT fibres. (a) Biofuel cell. At the anode, electrons are transferred from glucose to glucose oxidase (GOx) and from GOx to redox polymer (I) and from (I) to the CNT fibre. At the cathode, electrons are transferred from the CNT fibre to the redox polymer (II), from (II) to BOD and from BOD to oxygen. (b) CNT fibres before and (c) after removing PVA. Figure 1: Schematic of the biofuel cell and scanning electron micrographs of CNT fibres. ( a ) Biofuel cell. At the anode, electrons are transferred from glucose to glucose oxidase (GOx) and from GOx to redox polymer (I) and from (I) to the CNT fibre. At the cathode, electrons are transferred from the CNT fibre to the redox polymer (II), from (II) to BOD and from BOD to oxygen. ( b ) CNT fibres before and ( c ) after removing PVA. Full size image We show that a large improvement is observed in the electroreduction of oxygen to water in saline buffer on CNT fibres (CNFs) compared with a conventional CF, because the present electrodes combine radial transport and a large specific surface area. Under air and after several hours of operation, CNFs exhibit more than a tenfold higher performance. In addition, a glucose/oxygen BFC made with CNFs exhibit a power density of 740 μW cm −2 at +0.57 V in physiological conditions. Such power densities are one to two orders of magnitude higher than that of previous glucose/oxygen BFC, including recent ones made with GOx/BOD [20] , and fourfold higher than the power density obtained for a CF BFC. CNF preparation Several methods have been proposed to produce fibres solely comprised of nanotubes, but have never been used for bioelectrochemical purposes [25] , [26] , [27] , [28] , [29] . The porous CNF used in this study was formed by a coagulation spinning process that consists of injecting an aqueous CNT dispersion in a co-flowing stream of a polyvinyl alcohol (PVA) solution [30] . This process operated in water is continuous and scalable. The CNTs are first homogeneously dispersed in water by sonication using sodium dodecyl sulphate (SDS) as surfactant. The injection of the resulting dispersion in a rotating bath or in a co-axial pipe at a rate of 50 ml h −1 is carried out using a syringe needle. The CNTs coagulate on contacting the PVA solution because of bridging flocculation induced by adsorption of PVA chains at the CNT interface. The resultant composite fibres contain about 80 wt% PVA ( Fig. 1b ), which is then thermally decomposed by heating the fibres at 600 °C in an argon atmosphere. After this thermal treatment, the fibres become highly porous with a typical Brunauer-Emmett-Teller (BET) specific surface area of about 300 m 2 g −1 ( Fig. 1c ). Classical CFs, which are conventionally used for making microelectrodes, were tested for comparison. 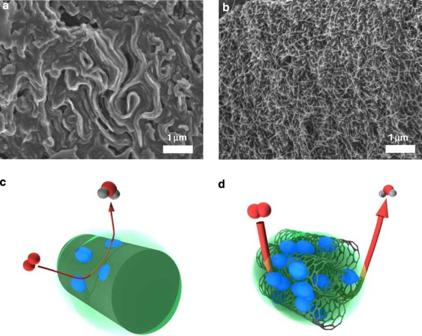Figure 2: Pictures and schematic of microelectrodes. SEM photographs of a carbon fibre (a) and a CNT fibre (b). Schematic representation of the oxygen reduction on the modified carbon fibre (c) and on the modified CNT fibre (d) (the green shade represents the redox polymer and the blue colour the enzymes). Figure 2 shows scanning electron micrographs of the cross-section of both the CF and CNT microwire. The advantage of the latter over the classical CF is apparent when examining the scanning electron microscope (SEM) images. In contrast to the non-porous CF, in which reduction of oxygen is only expected to occur at the external surface, the CNF is highly porous, with the pores being large enough to allow for easy permeation of the electrolyte and oxygen. By maximizing the porosity of the system, internal mass transfer limitations can be reduced [31] , [32] . Figure 2: Pictures and schematic of microelectrodes. SEM photographs of a carbon fibre ( a ) and a CNT fibre ( b ). Schematic representation of the oxygen reduction on the modified carbon fibre ( c ) and on the modified CNT fibre ( d ) (the green shade represents the redox polymer and the blue colour the enzymes). Full size image Electroreduction of oxygen CFs and CNFs were modified with a bioelectrocatalyst made of BOD, an oxygen-reducing enzyme, and a +0.34 V (versus Ag/AgCl) electron-conducting polymer, PAA-PVI-[Os(4,4′-dichloro-2,2′-bipyridine) 2 Cl] +/2+ . The resulting bioelectrocatalyst is an electrostatic adduct of the BOD, which is a polyanion at neutral pH, and of the electron-conducting polymer, which is a polycation. The formation of such an adduct prevents the phase separation of the enzyme and the polymer. The electron-conducting redox hydrogel obtained on crosslinking and hydration electrically 'connects' BOD redox centres to the electrode. It is permeated by water, oxygen and ions. Electron conduction results from the collisional electron transfer between reduced and oxidized redox centres tethered to the polymer backbone [33] , [34] . Because the rate of collisions increases with the mobility of the tethered redox centres, the greater their mobility the faster the electrons diffuse. High electron diffusivities are achieved in films that are only weakly crosslinked. However, weakly crosslinked films dissolve, or swell excessively, and are easily sheared off the electrodes. To prevent this shearing off of the electrocatalytic coatings and to maintain good mechanical properties, the adduct of the enzymes and their wires must still be crosslinked, even though this leads to a decrease in electronic conductivity and therefore of the current density [35] . The coating of electrodes consisted of 32.3 wt% BOD, 60.2 wt% redox polymer and 7.5 wt% poly(ethylene glycol) diglycidyl ether (PEGDGE). 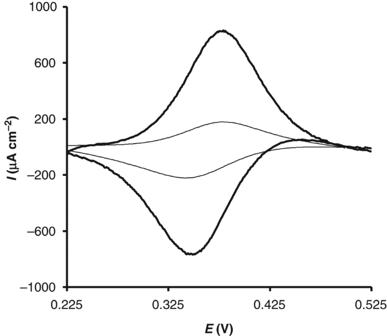Figure 3: Background subtracted cyclic voltammograms of the 'wired' BOD electrode. Dependence of current density (I) on voltage (V) for a CNT fibre (thick line) and a carbon fibre (thin line). Quiescent phosphate-buffered saline buffer, under argon atmosphere at 37 °C, 20 mV s−1, loading 170 μg. Figure 3 shows the background-subtracted cyclic voltammogram of the 'wired' BOD-coated CNF electrode (thick line) and CF electrode (thin line) under argon at 20 mV s −1 scan rate in a 20 mM phosphate buffer containing 0.14 M NaCl (pH 7.2) at 37 °C. At 1 mV s −1 scan rate, the voltammogram of the CNF exhibits an exactly symmetrical wave, with little separation (Δ E P =2 mV) of the oxidation and reduction peaks, typically indicative of a reversible surface-bound couple. The linear variation of peak height with scan rate confirms that the redox couple is surface confined. The width of the peak at half height, E whm , is 90 mV, close to the theoretical width of 90.6 mV for an ideal Nernstian one electron transfer reaction [10] . As shown in Fig. 3 , the voltammetric peaks at a rate of 20 mV s −1 are much narrower and closer to each other for the CNF than for the modified CF electrode. The voltage difference of the peaks is Δ E P =36 mV, compared with Δ E P =55 mV for the CF [36] , [37] . These distinctive features are ascribed to faster charge transport through the catalytic film made of CNTs. This is also evidenced by the decrease in the overpotential for oxygen reduction ( vide infra ). Interestingly, even though the exact same quantity of redox polymer was deposited on both electrode surfaces (that is, the same quantity of osmium centres), the oxidation and reduction current peaks of the CNF are fivefold higher. This suggests that not all redox centres are connected to the electrode surface of CFs. The increase in porosity provided by CNFs allows efficient access to a much higher fraction of redox polymer centres. The improvements are not only due to the porosity of the materials but also due to the conformations and electrical wiring of the enzymes and polymers to the electrode material. This is also why CNF electrodes exhibit much greater stability ( vide infra ). Figure 3: Background subtracted cyclic voltammograms of the 'wired' BOD electrode. Dependence of current density (I) on voltage (V) for a CNT fibre (thick line) and a carbon fibre (thin line). Quiescent phosphate-buffered saline buffer, under argon atmosphere at 37 °C, 20 mV s −1 , loading 170 μg. Full size image The current densities of a CF (thin line) and a CNF (thick line) modified with 'wired' BOD in a quiescent pH 7.2 along with 0.14 M NaCl, 20 mM phosphate buffer under air at 37 °C are compared in Fig. 4 . Under air and in quiescent solution, the CNF exhibits a fourfold higher current density than the conventional CF. The threshold for oxygen reduction is defined as the potential at which the electroreduction of oxygen starts [38] . It is 30 mV more oxidizing for the CNF compared with the CF. At +0.3 V/Ag/AgCl, oxygen is electroreduced at a current density of 1,570 μA cm −2 on the CNF, but at only 380 μA cm −2 on the CF. The overpotential, at any current density, is much lower for CNF electrodes and even better than platinum [14] , [39] . Under 1 atm oxygen and quiescent conditions, current densities >2.5 mA cm −2 are reached with CNFs. Such high current densities confirm that the porosity of CNFs offers an efficient solution to the intrinsic oxygen diffusion problem (present conditions: 0.2 mM concentration of oxygen in air-saturated saline buffer). The overpotential of three classes of electrodes is compared in 0.5 M H 2 SO 4 : a 6 μm diameter polished platinum cathode, a modified CF and a modified CNF. This comparison shows that the overpotential of the 'wired'-BOD/CNF cathode is much lower than that of the platinum fibre and is lower than that of the CF [14] , [39] . Thus, for example, for an overpotential of −0.31 V, oxygen was electroreduced to water at a current density that is 25-fold higher for the 'wired'-BOD cathode than for a polished platinum cathode in 0.5 M H 2 SO 4 . Moreover, the 'wired' BOD cathode operated in a physiological (20 mM phosphate, 0.14 M NaCl (pH 7.2)) buffer solution (phosphate-buffered saline), in which the platinum cathode would have rapidly corroded. 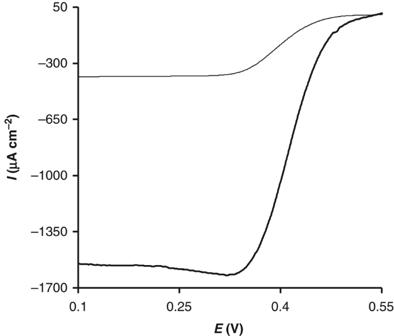Figure 4: Polarization curves for oxygen reduction. Dependence of current density (I) on voltage (V) for a modified CNT fibre electrode (thick line) and a modified carbon fibre electrode (thin line). Quiescent phosphate-buffered saline buffer, under air at 37 °C, 5 mV s−1, loading 170 μg. Figure 4: Polarization curves for oxygen reduction. Dependence of current density (I) on voltage (V) for a modified CNT fibre electrode (thick line) and a modified carbon fibre electrode (thin line). Quiescent phosphate-buffered saline buffer, under air at 37 °C, 5 mV s −1 , loading 170 μg. Full size image In addition, bioelectrocatalysts made of CNFs are more stable than their CF counterparts. It has been shown earlier that the incorporation of hydrophilic conductive graphite particles into highly crosslinked hydrogel produced a composite that could withstand the 2.4×10 −2 N m −2 shear stress resulting from the rotation of 3 mm diameter electrodes at 500 r.p.m. [40] . However, this also degraded the reversibility of the system. Incorporation of COOH-functionalized single-walled nanotubes in epoxy composites has also been shown to improve the mechanical performance of these composites and produced 40% enhancement in shear strength [41] . At a rotation rate of over 2,000 r.p.m., the CF that poised at +0.3 V/Ag/AgCl and at 37 °C loses 80% of its current density in 8 h. Under the same conditions, the CNF loses only 18% of its initial current density ( Fig. 5 ). After 8 h, the current of bioelectrocatalyst-modified CNFs is more than 10 times higher than that of the modified CF. This result shows that the bioelectrocatalyst is strengthened by CNFs through the formation of a strong three dimensional composite that can withstand shear stress >0.1×10 −2 N m −2 . To reach the same mechanical stability, more than 25% PEGDGE must be used with a modified CF, reducing the current density by more than 90%. 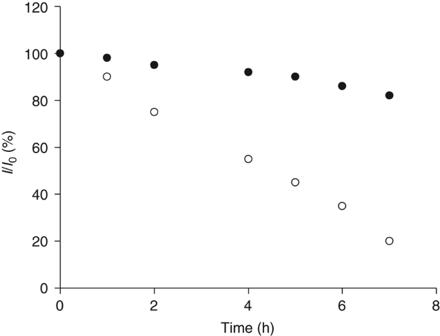Figure 5: Stability of the modified electrodes. Dependence of relative stability (%) on time (h) for a CNT fibre electrode (solid circles) and a carbon fibre (open circles). Phosphate-buffered saline buffer at 37 °C, +0.3 V/Ag/AgCl, under 1 atm oxygen and vigorous stirring, loading 170 μg. Figure 5: Stability of the modified electrodes. Dependence of relative stability (%) on time (h) for a CNT fibre electrode (solid circles) and a carbon fibre (open circles). Phosphate-buffered saline buffer at 37 °C, +0.3 V/Ag/AgCl, under 1 atm oxygen and vigorous stirring, loading 170 μg. Full size image Miniature membraneless glucose/oxygen BFC Finally, further evidence of interest of these fibres is shown by their use in a membraneless glucose/oxygen BFC operating in physiological conditions (pH 7.2, containing 20 mM phosphate, 0.14 M NaCl at 37 °C) [11] , [16] , [24] , [42] , [43] , [44] , [45] , [46] , [47] . In a glucose/oxygen BFC, glucose is electrooxidized at the anode, Oxygen is reduced to water at the cathode, resulting in the net bioelectrochemical power-generating reaction The cell used in this study [48] is made of two 7 μm diameter, 2 cm long, bioelectrocatalyst-coated CFs or CNFs. The carbon and CNF cathodes were those described above, with their characterizations as shown in Figure 3 . Both anode types were made of GOx from Aspergillus niger and a corresponding redox polymer [36] , [37] , [48] . 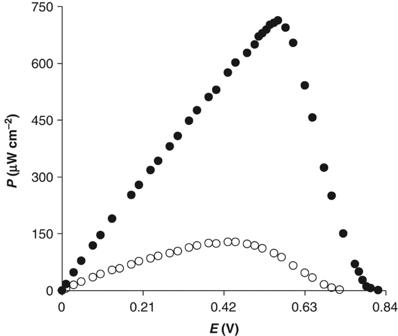Figure 6: Power density curves. Dependence of power density (P) on operating voltage (V) for a biofuel cell made with carbon fibre (open circles) and CNT fibre (solid circles) in a quiescent phosphate-buffered saline buffer, under air, 15 mM glucose at 37 °C, loading 226 μg. The dependence of power density on the operating voltage of the assembled CNT (black circles) and of the assembled CF (empty circles) BFCs is shown in Figure 6 in a quiescent air 20 mM phosphate buffer solution containing 0.14 M NaCl at 37 °C. The curves exhibit the typical shape of the BFC power curve with three regions corresponding to (1) the activation losses at low current density governed by the activation overpotential that arises from the kinetics of electron transfer reactions; (2) the ohmic losses that arise from the resistance of BFC and depend on the materials used and the interface between polymers/enzymes and electrodes; and (3) the concentration polarization at high current density that depends on mass transport [49] . At 15 mM glucose concentration, the maximum power density for the CNT BFC is 740 μW cm −2 at a voltage of +0.57 V, which is fourfold higher than the power density obtained for the CF BFC (180 μW cm −2 at +0.45 V). It is also almost two orders of magnitudes larger than the power of a recently reported BFC using GOx and BOD as bioelectrocatalysts [20] . The open-circuit voltage (OCV) for the CF BFC was +0.73 V, whereas it was +0.83 V for the CNT BFC. The OCV provides a measure of the maximum voltage associated with the BFC, which depends on enzymes, polymers and electrode materials. In an ideal case, OCV should be equal to the difference of the thermodynamic potentials of the involved redox species. The significant increase in OCV of the CNT glucose/oxygen BFC reflects a more efficient electrical wiring of enzymes to the CNT electrode surface, compared with the CF BFC, because of a poorer electronic connection to the electrode. The better electrical connection to the CNT results in lower energetic barriers for electron transfer from enzymes to the electrode. This also explains why the maximum of the operating voltage of the BFC is observed at a higher voltage for CNFs, compared with CFs. Figure 6: Power density curves. Dependence of power density (P) on operating voltage (V) for a biofuel cell made with carbon fibre (open circles) and CNT fibre (solid circles) in a quiescent phosphate-buffered saline buffer, under air, 15 mM glucose at 37 °C, loading 226 μg. Full size image Because the sizes of microelectronic circuits and sensors are constantly reduced, the size of the low-power sensor-transmitter packages for physiological research and medicine becomes limited by the size of their power source. Miniature membraneless glucose/oxygen BFCs may power such devices. For example, such BFC would power a subcutaneously implanted, continuous glucose monitor for diabetes management. Operating such devices at a high-power density requires a large number of enzymes efficiently wired to the anode or the cathode and a fast enzyme turnover rate. It also requires that mass transport of products and reactants to/from electrodes should not be limited by diffusion and that the size of the BFC be small enough to be eventually implanted. The engineering of new porous and hybrid microfibres made of oriented and biofunctionalized CNTs addresses these challenges. CNFs are highly porous, with pores being large enough to allow permeation of the electrolyte without inducing unwanted concentration polarization, such as localized pH gradients that could affect enzyme activity. After 150 h of operation, the cell only lost 20% of its power density. Compared with CFs, the use of CNT electrodes has five main advantages: (1) the high specific surface that yields a higher power density; (2) more efficient connections of redox polymers and enzymes to electrode materials; (3) porosity that allows permeation of the species without unwanted polarization of concentrations; (4) reduction of the overpotential required for glucose electrooxidation and oxygen electroreduction; and (5) stabilization of bioelectrocatalysts. Because of the selectivity of our bioelectrocatalysts and the use of CNFs, we succeeded in achieving a high-power density with miniaturized (0.0044 mm 2 ) and membraneless BFC. The membraneless BFC generated 740 μW cm −2 at +0.57 V, exceeding by far the power density obtained for CF membraneless BFCs. Recently, Sakai et al . [24] also reported a high-power glucose/oxygen membrane BFC generating 1.45 mW cm −2 at +0.3 V, which is twice as high as the power generated by the present BFCs. However, to reach such power densities, membranes were implemented to separate anodic and cathodic compartments because of the use of soluble redox mediators. Even though such BFCs exhibit a high-power density, they are not designed for the same applications and implantable devices. Indeed, the use of membranes and separation of anodic and cathodic compartments prevent extreme miniaturization down to micron-sized devices. In summary, the adequate engineering of CNTs into microwires can open up new synthetic routes for novel electrodes that overcome mass transport limitations and provide high specific areas. The current density can be enhanced by increasing the surface area through CNTs while maintaining high rates of species transport and excellent structural stability. The obtained electrodes exhibit properties that largely exceed the properties of currently available electrodes made of CFs. This was shown through the electroreduction of oxygen to water and through the construction of a high-power, miniature, membraneless BFC. Under air and in a quiescent solution, a modified CNT microwire functions more than ten times better than a conventional CF. The maximum power density of a CNT BFC is fourfold higher than the power density obtained for a CF BFC. In addition, the overpotential, at any current density, is lower than that observed at platinum. Finally, apart from its straightforward interest for electrochemistry, because of the improved properties in terms of current density, reactivity and stability, we expect this novel class of electrodes to be a starting point for the elaboration of various high-performance biosensors and electrochemical devices. Chemicals BOD (EC 1.3.3.5) from Trachyderma tsunodae was purchased from Amano and purified as described previously [14] . GOx from Aspergillus niger (EC 1.1.3.4, 208 U mg −1 ) was purchased from Fluka (Sigma-Aldrich) and purified as previously described [50] . Poly(ethylene glycol) (MW 400) diglycidyl ether(PEGDGE) was purchased from Polysciences, poly(vinyl alcohol) (PVA, MW 195,000) from Kuraray Europe GmbH and SDS from Aldrich and used as received. The synthesis of the BOD-wiring redox polymer PAA-PVI-[Os(4,4′-dichloro-2,2′-bipyridine) 2 Cl] +/2+ and that of the GOX-wiring polymer PVP-[Os( N , N ′-alkylanated-2,2′bi-imidazole) 3 ] 2+/3 were reported earlier [35] , [36] . Single-walled CNTs produced from a high-pressure CO disproportionation (HiPco) process were purchased from Carbon Nanotech. All aqueous solutions were prepared with Millipore ultrapure water. Instrumentation Measurements were performed using a potentiostat (CH Instruments, model CHI 760C) and a dedicated computer. A platinum spiral wire was used as counter electrode and all potentials were referred to a Ag/AgCl (3 M KCl) electrode. Either CNFs or CFs were used as the working electrode. The morphology of the CNFs and CFs was characterized by a field emission scanning electron microscope (Model JSM-6700F, JEOL) operated at a voltage of 5.0 kV. The sample was prepared by fixing the CNF fibre or the CF on a SEM stage using carbon tape. Fibre synthesis CNTs were first purified by acid treatment before producing fibres. Typically, 250 mg of CNTs was heated at 200 °C in an oven for 8 h, then placed in a flask. A concentration of 1 l HCl (37%, v/v) was poured into the flask and incubated for 4 h under agitation. The colour of the solution became yellow because of the dissolution of Fe 3+ ions. After suction filtration, the tubes were washed several times with deionized water. They were then lyophilized. The CNFs are made by a particle coagulation spinning process. CNTs were dispersed and stabilized in aqueous solutions of SDS (1.0 wt%). Homogeneous dispersions were achieved by sonication. A relatively concentrated aqueous CNT suspension (0.3 wt%) is injected through a cylindrical syringe into the co-flowing stream of a coagulating bath containing PVA solution (5 wt%). As a result, CNTs aggregate and form gel-like fibres. The gel fibres are washed several times with pure water to remove most of the surfactant and some fraction of PVA. They are then pulled out of water, dried and collated into a composite CNT–PVA fibre. As-produced CNFs consist of an interconnected network of PVA chains and CNTs. They exhibit a high toughness. However, they are not suitable as such for electrochemical applications. Indeed, PVA limits the porosity of fibres and the access to the CNT interface. This is why fibres were heated at a temperature of 600 °C for 2 h under argon atmosphere to completely remove the PVA. After this thermal treatment, fibres are electrically conductive and only composed of CNT without any additives or binders. They exhibit a high porosity and are therefore suitable for electrochemical applications. The SEM images of the CNF before and after removing PVA are shown below. The diameter of the fibres can be controlled by the flows in the spinning process. In the present experiments, the diameter of the investigated fibres was 9.5 μm. The CFs used for comparisons have a diameter of 7 μm. Electrode preparation The CNF electrode was synthesized as follows: (1) a single fibre was placed in a 1 mm polycarbonate groove. (2) One end of the fibre was fixed by epoxy and the other end was electrically connected to a copper wire with conductive carbon paint. (3) The carbon paint was allowed to dry and then insulated with a layer of epoxy. (4) Before coating the bioelectrocatalysts, the CNF was made hydrophilic by plasma oxidation (1 torr oxygen plasma, 20 min). Unless stated otherwise, the electrochemical experiments were carried out in air under quiescent conditions and in a 20 mM phosphate buffer containing 0.14 M NaCl (pH 7.2) at 37 °C. Fibre properties and electrochemical characterizations The CNFs are electrically conductive and exhibit a conductivity of 50 S cm −1 , as measured by a Keithley 2000 multimeter between two silver paint connections. All electrochemical data are normalized by the geometric area and volume of the fibres. The CNF electrochemical capacitance measured in a 1 M NaCl aqueous solution is about 20 F cm −3 . BET surface area was measured by nitrogen adsorption–desorption experiments at 77.4 K, as previously reported for similar fibres [51] . It is about 300 m 2 g −1 . Increasing the porosity of an electrode material is a key to increase its electroactive surface area. Nevertheless, a direct determination of the actual microscopic area of a microelectrode from electrochemical measurements is not straightforward. Indeed, features of roughness smaller than the diffusion length tend to be averaged within the diffusion field [10] . This is why comparisons between electrochemical capacitance and BET surface area should be taken with some caution. How to cite this article: Gao, F. et al . Engineering hybrid nanotube wires for high-power biofuel cells. Nat. Commun. 1:2 doi: 10.1038/ncomms1000 (2010).